Leucine-rich repeat kinase LRRK1 regulates endosomal trafficking of the EGF receptor Activation of the epidermal growth factor receptor (EGFR) not only initiates multiple signal-transduction pathways, including the MAP kinase (MAPK) pathway, but also triggers trafficking events that relocalize receptors from the cell surface to intracellular endocytic compartments. In this paper, we demonstrate that leucine-rich repeat kinase LRRK1, which contains a MAPKKK-like kinase domain, forms a complex with activated EGFR through an interaction with Grb2. Subsequently, LRRK1 and epidermal growth factor (EGF) are internalized and co-localized in early endosomes. LRRK1 regulates EGFR transport from early to late endosomes and regulates the motility of EGF-containing early endosomes in a manner dependent on its kinase activity. Furthermore, LRRK1 serves as a scaffold facilitating the interaction of EGFR with the endosomal sorting complex required for transport-0 complex, thus enabling efficient sorting of EGFR to the inner vesicles of multivesicular bodies. Our findings provide the first evidence that a MAPKKK-like protein regulates the endosomal trafficking of EGFR. Binding of epidermal growth factor (EGF) to its cell surface receptor (EGFR) results in the activation of numerous cell signalling pathways essential for cellular proliferation, survival and differentiation. Activation of EGFR also initiates events leading to its endocytosis [1] , [2] . Receptors, once internalized, are delivered to the endosomal system, from where they are either recycled to the cell surface or sorted to lysosomes for degradation [3] , [4] , [5] . Endocytic trafficking serves as an important determinant of the intensity and duration of EGFR signalling. Recent studies have shown that the endosomal sorting complexes required for transport, ESCRT-0, -I, -II and -III, are involved in the endosomal sorting of ubiquitinated EGFR to lysosomes through multivesicular bodies (MVBs) [6] , [7] , [8] , [9] , [10] . The ESCRT-0 complex, which is composed of hepatocyte growth factor-regulated substrate (Hrs) and signal-transducing adaptor molecule (STAM), is believed to initiate the process by which EGFR is targeted to lysosomes at the early endosome stage. This targeting involves the clustering of ubiquitinated EGFR underneath a clathrin microdomain by recruiting the ESCRT-I complex to the surface of endosomes. Binding of ESCRT-I to the surface of endosomes leads to the sequential recruitment of ESCRT-II and ESCRT-III complexes. These complexes function sequentially in the formation of MVB vesicles and in the sorting of EGFR into the MVB pathway. Thus, the recognition of EGFR by the ESCRT-0 complex is a critical step in the sorting of EGFR to lysosomes. Human LRRK1 and LRRK2 belong to the ROCO family of proteins and contain a Roc (Ras in complex proteins) domain together with a MAPKKK-like kinase domain and several protein–protein interaction domains. Recently, LRRK2 has been reported to be involved in the pathogenesis of familial Parkinson's disease [11] , [12] . However, the functions of LRRK1 and LRRK2 remain unknown. In this study, we identified Grb2, which is known to be essential for EGFR signalling and endocytosis [1] , [13] , [14] , [15] , [16] , as an LRRK1-interacting protein. We demonstrate that LRRK1 participates in the intracellular trafficking of EGFR through an interaction with Grb2. Our findings indicate that LRRK1 regulates transport and sorting of EGFR in a manner dependent on and independent of its kinase activity, respectively. LRRK1 forms a complex with activated EGFR via Grb2 To investigate the physiological roles of LRRK1, we attempted to identify molecules with which it interacts. We used liquid chromatography-coupled tandem mass spectrometry (LC–MS/MS) [17] , and identified multiple peptides ( Supplementary Table S1 ). Among the proteins identified, we focused on the Grb2 protein. To confirm the association between LRRK1 and Grb2, COS7 cells were co-transfected with Flag-LRRK1 and HA-Grb2. 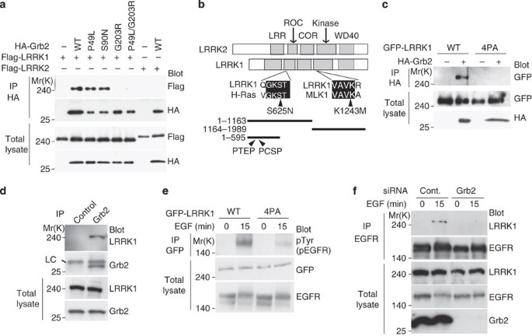Figure 1: LRRK1 forms a complex with EGFR via Grb2 in response to EGF stimulation. (a) Interaction of LRRK1 with Grb2. COS7 cells were co-transfected with Flag-LRRK1, Flag-LRRK2 and HA-Grb2 (wild type (WT), P49L, S90N, G203R and P49L/G203R mutants), as indicated. Complex formation was detected by immunoprecipitation (IP) with anti-HA antibodies, followed by immunoblotting (Blot) with anti-Flag antibodies. (b) Comparison of LRRK1 and LRRK2 structures. Schematic diagrams of human LRRK1 and LRRK2 proteins are shown. Domains are shown as follows: leucine-rich repeats (LRR), a Roc domain, a Cor domain, a MAPKKK-like kinase domain and WD40 repeats. The sequence alignment of LRRK1 and H-Ras in the Roc domain and of LRRK1 and mixed-lineage kinase 1 (MLK1) in the kinase domain are shown. Identical residues are highlighted with black shading. Arrowheads indicate amino-acid substitutions used in this study. Deletion constructs of LRRK1 are shown below. Two PXXP motifs within LRRK1(1–595) are shown by the arrowheads. (c) Effect of the 4PA mutation on the interaction of LRRK1 with Grb2. COS7 cells were co-transfected with GFP-LRRK1 (wild type and the 4PA mutant) and HA-Grb2, as indicated. Complex formation was detected by immunoprecipitation (IP) with anti-HA antibodies, followed by immunoblotting (Blot) with anti-GFP antibodies. (d) Interaction of endogenous LRRK1 with endogenous Grb2. Complex formation in HEK293 cells was detected by immunoprecipitation (IP) with anti-Grb2 antibodies, followed by immunoblotting (Blot) with anti-LRRK1 antibodies. LC, light chain. (e) Effect of the 4PA mutation on the interaction of LRRK1 with activated EGFR. COS7 cells were transfected with GFP-LRRK1 (wild type and the 4PA mutant). After 16 h of serum starvation, cells were stimulated with 100 ng per ml of EGF. Complex formation was detected by immunoprecipitation (IP) with anti-GFP antibodies, followed by immunoblotting (Blot) with anti-phospho-tyrosine (pTyr) antibodies. (f) Interaction of endogenous LRRK1 with endogenous EGFR. HEK293 cells treated with control or Grb2 siRNA were serum starved and stimulated with 100 ng per ml of EGF. Complex formation was detected by immunoprecipitation (IP) with anti-EGFR antibodies, followed by immunoblotting (Blot) with anti-LRRK1 antibodies. As seen in Figure 1a , Flag-LRRK1 associated with HA-Grb2. This association was specific for LRRK1, because LRRK2 did not interact with Grb2 ( Fig. 1a ). Figure 1: LRRK1 forms a complex with EGFR via Grb2 in response to EGF stimulation. ( a ) Interaction of LRRK1 with Grb2. COS7 cells were co-transfected with Flag-LRRK1, Flag-LRRK2 and HA-Grb2 (wild type (WT), P49L, S90N, G203R and P49L/G203R mutants), as indicated. Complex formation was detected by immunoprecipitation (IP) with anti-HA antibodies, followed by immunoblotting (Blot) with anti-Flag antibodies. ( b ) Comparison of LRRK1 and LRRK2 structures. Schematic diagrams of human LRRK1 and LRRK2 proteins are shown. Domains are shown as follows: leucine-rich repeats (LRR), a Roc domain, a Cor domain, a MAPKKK-like kinase domain and WD40 repeats. The sequence alignment of LRRK1 and H-Ras in the Roc domain and of LRRK1 and mixed-lineage kinase 1 (MLK1) in the kinase domain are shown. Identical residues are highlighted with black shading. Arrowheads indicate amino-acid substitutions used in this study. Deletion constructs of LRRK1 are shown below. Two PXXP motifs within LRRK1(1–595) are shown by the arrowheads. ( c ) Effect of the 4PA mutation on the interaction of LRRK1 with Grb2. COS7 cells were co-transfected with GFP-LRRK1 (wild type and the 4PA mutant) and HA-Grb2, as indicated. Complex formation was detected by immunoprecipitation (IP) with anti-HA antibodies, followed by immunoblotting (Blot) with anti-GFP antibodies. ( d ) Interaction of endogenous LRRK1 with endogenous Grb2. Complex formation in HEK293 cells was detected by immunoprecipitation (IP) with anti-Grb2 antibodies, followed by immunoblotting (Blot) with anti-LRRK1 antibodies. LC, light chain. ( e ) Effect of the 4PA mutation on the interaction of LRRK1 with activated EGFR. COS7 cells were transfected with GFP-LRRK1 (wild type and the 4PA mutant). After 16 h of serum starvation, cells were stimulated with 100 ng per ml of EGF. Complex formation was detected by immunoprecipitation (IP) with anti-GFP antibodies, followed by immunoblotting (Blot) with anti-phospho-tyrosine (pTyr) antibodies. ( f ) Interaction of endogenous LRRK1 with endogenous EGFR. HEK293 cells treated with control or Grb2 siRNA were serum starved and stimulated with 100 ng per ml of EGF. Complex formation was detected by immunoprecipitation (IP) with anti-EGFR antibodies, followed by immunoblotting (Blot) with anti-LRRK1 antibodies. Full size image Grb2 contains a single SH2 domain flanked by two SH3 domains [14] . We examined whether the SH2 or SH3 domain is required for interaction with LRRK1. Mutations in the amino (N)-terminal SH3 (P49L) or SH2 (S90N) domain of Grb2 had no effect on its interaction with LRRK1 ( Fig. 1a ). In contrast, a mutation in its carboxy (C)-terminal SH3 domain (G203R) resulted in the loss of detectable binding to LRRK1 ( Fig. 1a ). Thus, interaction of Grb2 with LRRK1 requires the C-terminal SH3 domain of Grb2. We next examined which region of LRRK1 is required for its association with Grb2. We constructed several deletion mutants of LRRK1 ( Fig. 1b ) and analysed their binding to Grb2. C-terminal-deleted mutants LRRK1(1–1163) and LRRK1(1–595), but not the N-terminal-deleted mutant LRRK1(1164–1989), bound to Grb2 ( Supplementary Fig. S1 ). It is known that the SH3 domain of Grb2 binds to the proline-based motif PXXP [14] . As the LRRK1(1–595) fragment contains two PXXP motifs, which are located at residues 88–91 and 119–122 ( Fig. 1b ), we examined whether these sites are responsible for Grb2 association. We found that mutation of the Pro residues in both PXXP motifs to Ala (mutant LRRK1(P88A/P91A/P119A/P122A); LRRK1(4PA)) eliminated binding to Grb2 ( Fig. 1c ). These results indicate that LRRK1 associates with Grb2 through an interaction between the PXXP motifs of LRRK1 and the C-terminal SH3 domain of Grb2. Using a polyclonal anti-LRRK1 antibody that we generated ( Supplementary Fig. S2 ), we also investigated the interaction of endogenously expressed LRRK1 and Grb2. We found that endogenous LRRK1 was able to associate with endogenous Grb2 in a ligand-independent manner ( Fig. 1d ). Because Grb2 functions as an adaptor protein facilitating the association of several factors with activated EGFR [14] , [15] , we examined whether LRRK1 forms a complex with EGFR in response to EGF stimulation. COS7 cells were transfected with GFP-LRRK1. We found that GFP-LRRK1 bound to EGFR in a stimulus-dependent manner ( Fig. 1e ). In contrast, the Grb2-binding-defective mutant GFP-LRRK1(4PA) was unable to associate with EGFR after EGF stimulation ( Fig. 1e ), suggesting that Grb2 mediates the interaction between LRRK1 and EGFR. We also found that endogenous LRRK1 was able to form a complex with EGFR following EGF stimulation ( Fig. 1f ). Furthermore, when cells were depleted of Grb2 by transfection with small interfering RNA (siRNA), LRRK1 was unable to interact with EGFR in response to EGF stimulation, regardless of where endogenous or overexpressed LRRK1 was used ( Fig. 1f ; Supplementary Fig. S3 ). Taken together, these results demonstrate that LRRK1 forms a complex with EGFR in response to EGF stimulation in a Grb2-dependent manner. LRRK1 co-localizes with EGF in early endosomes To investigate the role of LRRK1 in EGFR signalling, we examined the subcellular localization of LRRK1. Because our polyclonal anti-LRRK1 antibody did not provide a sensitive enough detection of the endogenous protein by immunostaining, we used an epitope-tagged LRRK1. We expressed GFP-LRRK1 in HeLa cells and assessed LRRK1 localization by immunofluorescence under basal and EGF-stimulated conditions, together with a fluorescently labelled rhodamine-conjugated EGF (EGF-Rh). LRRK1 was diffusely distributed in cells not treated with EGF-Rh ( Fig. 2a ). When cells were stimulated with EGF-Rh for 15 min, GFP-LRRK1 became distributed in a fine, punctate pattern that co-localized with EGF-Rh. A large portion of GFP-LRRK1 overlapped with the early endosomal marker autoantigen 1 (EEA1) receptor ( Fig. 2b ; Supplementary Fig. S4 ). 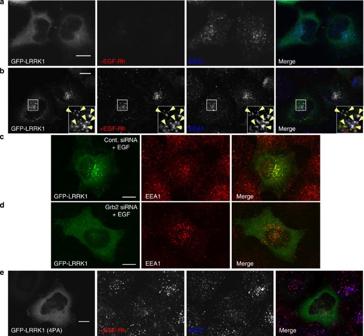Figure 2: LRRK1 co-localizes with EGF in early endosomes. (a,b) Co-localization of LRRK1 with EGF in EEA1-labelled early endosomes. HeLa cells were transfected with GFP-LRRK1. After 16 h of serum starvation, cells were incubated without (a) or with (b) 50 ng per ml of EGF-Rh (red) for 45 min at 4°C, followed by warming for 15 min at 37°C, and stained with anti-EEA1 antibodies (blue). All cells were imaged by confocal microscopy. The boxed regions are magnified in insets. Examples of co-localization of GFP-LRRK1, EGF-Rh and EEA1 are indicated with arrowheads (Supplementary Fig. S4). Scale bar, 10 μm. (c,d) Effect of Grb2 depletion on LRRK1 localization in early endosomes. HeLa S3 cells treated with control (c) or Grb2 siRNA (d) were transfected with GFP-LRRK1. After 16 h of serum starvation, cells were stimulated with 100 ng per ml of EGF for 15 min. The cells were fixed, stained with anti-EEA1 antibodies and imaged by confocal microscopy. Yellow colour in the merged images indicates co-localization. Scale bar, 10 μm. (e) Effect of 4PA mutation on LRRK1 localization. HeLa cells were transfected with GFP-LRRK1(4PA). After 16 h of serum starvation, cells were incubated with 50 ng per ml of EGF-Rh (red) for 45 min at 4°C, followed by warming for 15 min at 37°C, and stained with anti-EEA1 antibodies (blue). All cells were imaged by confocal microscopy. Scale bar, 10 μm. Figure 2: LRRK1 co-localizes with EGF in early endosomes. ( a , b ) Co-localization of LRRK1 with EGF in EEA1-labelled early endosomes. HeLa cells were transfected with GFP-LRRK1. After 16 h of serum starvation, cells were incubated without ( a ) or with ( b ) 50 ng per ml of EGF-Rh (red) for 45 min at 4°C, followed by warming for 15 min at 37°C, and stained with anti-EEA1 antibodies (blue). All cells were imaged by confocal microscopy. The boxed regions are magnified in insets. Examples of co-localization of GFP-LRRK1, EGF-Rh and EEA1 are indicated with arrowheads ( Supplementary Fig. S4 ). Scale bar, 10 μm. ( c , d ) Effect of Grb2 depletion on LRRK1 localization in early endosomes. HeLa S3 cells treated with control ( c ) or Grb2 siRNA ( d ) were transfected with GFP-LRRK1. After 16 h of serum starvation, cells were stimulated with 100 ng per ml of EGF for 15 min. The cells were fixed, stained with anti-EEA1 antibodies and imaged by confocal microscopy. Yellow colour in the merged images indicates co-localization. Scale bar, 10 μm. ( e ) Effect of 4PA mutation on LRRK1 localization. HeLa cells were transfected with GFP-LRRK1(4PA). After 16 h of serum starvation, cells were incubated with 50 ng per ml of EGF-Rh (red) for 45 min at 4°C, followed by warming for 15 min at 37°C, and stained with anti-EEA1 antibodies (blue). All cells were imaged by confocal microscopy. Scale bar, 10 μm. Full size image We next analysed the ability of Grb2 to affect the intracellular localization of LRRK1 in EGF-stimulated cells. When Grb2 was depleted from HeLa S3 cells using siRNA, EGF-induced localization of LRRK1 in EEA1-positive early endosomes was greatly decreased ( Fig. 2c,d ; Supplementary Fig. S5a ). This suggests that Grb2 is required for the EGF-induced translocation of LRRK1 to early endosomes. Consistent with this, LRRK1(4PA), which is defective for Grb2 binding, failed to localize to early endosomes in response to EGF stimulation ( Fig. 2e ; Supplementary Fig. S5b ). Thus, EGF-induced localization of LRRK1 to early endosomes is dependent on Grb2-mediated complex formation with activated EGFR. LRRK1 regulates EGFR transport from early to late endosomes Given the EGF-dependent association of LRRK1 with the early endosome, we reasoned that LRRK1 might function by affecting the endocytic trafficking of EGFR. To test this idea, we monitored the endocytic movement of EGF in cells depleted of LRRK1 by siRNA. HeLa S3 cells incubated with LRRK1 siRNA had a much lower expression of LRRK1 ( Supplementary Fig. S6 ). HeLa S3 cells treated with control or LRRK1 siRNA were stimulated with fluorescent EGF (Alexa 647-EGF) briefly, followed by washing to remove labelled EGF from the medium. Under these conditions, the fluorescence detected in cells was due to endocytosed EGFR bound to labelled growth factor. In LRRK1-depleted cells, the initial localization of EGF to clathrin-coated pits occurred normally, similar to control cells ( Supplementary Fig. S7 ). Thus, depletion of LRRK1 has little obvious effect on the internalization of EGF/EGFR. Because it is known that Rab5 and Rab7 primarily associate with early and late endosomes, respectively, we coexpressed GFP-Rab5 and DsRed-Rab7 in HeLa S3 cells to visualize early and late endosomes. In this experiment, we used the monomer version of DsRed. Most of the Rab5-positive endosomes were distributed in the cell periphery, whereas Rab7-positive endosomes were more common in the perinuclear region ( Fig. 3a–d ). In control siRNA-transfected cells, at 10 min after a brief pulse of Alexa 647-EGF stimulation, most of the EGF was found in early endosomes, as evidenced by their co-localization with Rab5 ( Fig. 3a,e ; Supplementary Fig. S8a ). After 15 min, EGF dissociated from the early endosomes, as illustrated by decreased co-localization with Rab5. Remarkably, this decreased co-localization with Rab5 was accompanied by an increase in the co-localization with Rab7 ( Fig. 3b,e and f ; Supplementary Fig. S8b ), suggesting the progression of EGFR to the late-endosomal compartments. In LRRK1-depleted cells, the early endosomal localization of EGF occurred normally, as in control cells ( Fig. 3c,e ; Supplementary Fig. S8c ). However, after 15 min of stimulation, Alexa 647-EGF remained associated with Rab5-positive structures and Rab7 co-localization did not increase ( Fig. 3d–f ; Supplementary Fig. S8d ). This suggests that the transport of EGFR towards late endosomes is inhibited in LRRK1-deficient cells. Thus, LRRK1 is required for the progression of EGFR from early to late endosomes. 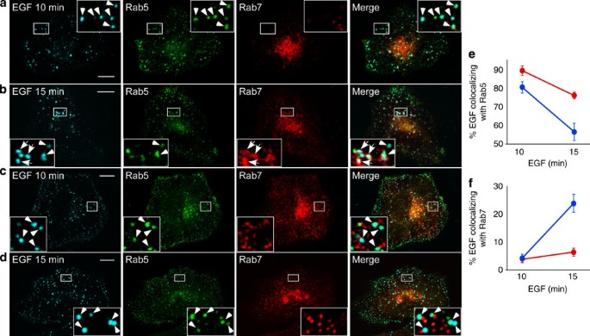Figure 3: Depletion of LRRK1 inhibits EGFR transport from early to late endosomes. (a,b) HeLa S3 cells treated with control siRNA were co-transfected with GFP-Rab5 and DsRed-Rab7. After 16 h of serum starvation, cells were stimulated with 100 ng per ml of Alexa 647-EGF for 3 min at 37°C, followed by washing to remove labelled EGF from the medium. The cells were fixed at 10 min (a) and 15 min (b) after the initial exposure to Alexa 647-EGF and imaged by confocal microscopy. The boxed regions are magnified in insets. Arrowheads and arrows indicate co-localization of Alexa 647-EGF with GFP-Rab5 and DsRed-Rab7, respectively (Supplementary Fig. S8). Scale bar, 10 μm. (c,d) Effect of LRRK1 depletion on EGFR transport from early to late endosomes. HeLa S3 cells treated with LRRK1 siRNA (Stealth#1) were co-transfected with GFP-Rab5 and DsRed-Rab7. After 16 h of serum starvation, cells were stimulated with 100 ng per ml of Alexa 647-EGF for 3 min at 37°C, followed by washing to remove labelled EGF from the medium. The cells were fixed at 10 min (c) and 15 min (d) after the initial exposure to Alexa 647-EGF and imaged by confocal microscopy. The boxed regions are magnified in insets. Arrowheads indicate co-localization of Alexa 647-EGF with GFP-Rab5 (Supplementary Fig. S8). Scale bar, 10 μm. (e,f) Quantification of co-localization of EGFR with Rab5 (e) and Rab7 (f). Cells treated with control (blue) or LRRK1 siRNA (Stealth#1) (red) were co-transfected with GFP-Rab5 and DsRed-Rab7. After 16 h of serum starvation, cells were stimulated with 100 ng per ml of Alexa 647-EGF for 3 min at 37°C, followed by washing to remove labelled EGF from the medium. The cells were fixed at 10 min and 15 min after the initial exposure to Alexa 647-EGF. Data are presented as percentages of Rab5-labelled (e) or Rab7-labelled (f) Alexa647-EGF-containing vesicles out of the total number of Alexa647-EGF-containing vesicles per cell. Values reflect the mean s.d. of three independent experiments, with an average of ten cells scored per experiment. Figure 3: Depletion of LRRK1 inhibits EGFR transport from early to late endosomes. ( a , b ) HeLa S3 cells treated with control siRNA were co-transfected with GFP-Rab5 and DsRed-Rab7. After 16 h of serum starvation, cells were stimulated with 100 ng per ml of Alexa 647-EGF for 3 min at 37°C, followed by washing to remove labelled EGF from the medium. The cells were fixed at 10 min ( a ) and 15 min ( b ) after the initial exposure to Alexa 647-EGF and imaged by confocal microscopy. The boxed regions are magnified in insets. Arrowheads and arrows indicate co-localization of Alexa 647-EGF with GFP-Rab5 and DsRed-Rab7, respectively ( Supplementary Fig. S8 ). Scale bar, 10 μm. ( c , d ) Effect of LRRK1 depletion on EGFR transport from early to late endosomes. HeLa S3 cells treated with LRRK1 siRNA (Stealth#1) were co-transfected with GFP-Rab5 and DsRed-Rab7. After 16 h of serum starvation, cells were stimulated with 100 ng per ml of Alexa 647-EGF for 3 min at 37°C, followed by washing to remove labelled EGF from the medium. The cells were fixed at 10 min ( c ) and 15 min ( d ) after the initial exposure to Alexa 647-EGF and imaged by confocal microscopy. The boxed regions are magnified in insets. Arrowheads indicate co-localization of Alexa 647-EGF with GFP-Rab5 ( Supplementary Fig. S8 ). Scale bar, 10 μm. ( e , f ) Quantification of co-localization of EGFR with Rab5 ( e ) and Rab7 ( f ). Cells treated with control (blue) or LRRK1 siRNA (Stealth#1) (red) were co-transfected with GFP-Rab5 and DsRed-Rab7. After 16 h of serum starvation, cells were stimulated with 100 ng per ml of Alexa 647-EGF for 3 min at 37°C, followed by washing to remove labelled EGF from the medium. The cells were fixed at 10 min and 15 min after the initial exposure to Alexa 647-EGF. Data are presented as percentages of Rab5-labelled ( e ) or Rab7-labelled ( f ) Alexa647-EGF-containing vesicles out of the total number of Alexa647-EGF-containing vesicles per cell. Values reflect the mean s.d. of three independent experiments, with an average of ten cells scored per experiment. Full size image LRRK1 regulates the motility of EGF-early endosomes Because maturation of early to late endosomes is accompanied by the movement of endosomes towards the cell centre [18] , [19] , [20] , we examined the effect of LRRK1 knockdown on the movement of EGF-containing early endosomes. Using time-lapse confocal fluorescence microscopy, movement of EGF-containing early endosomes was followed in cells expressing GFP-Rab5 at 15 min after a brief pulse of Alexa647-EGF. In addition to short-range movement, long-range rapid movement of EGF-positive early endosomes from the periphery to the centre was frequently observed ( Fig. 4a,b ). When LRRK1 was knocked down by siRNA, long-range rapid movement of EGF-containing early endosomes was remarkably disrupted ( Fig. 4c,d ). In control cells, 39.7% of GFP-Rab5- and Alexa 647-EGF-double-positive endosomes moved more than 3.0 μm during the imaging time (35 s), but this fraction decreased to only 2.4% in LRRK1-depleted cells ( Fig. 4e ). We further confirmed this effect of knocking down LRRK1 on the frequency of long-range movement of EGF using a different LRRK1 siRNA in different HeLa cell lines ( Supplementary Fig. S9 ). These observations suggest that LRRK1 is required for the motility of EGF-containing early endosomes. 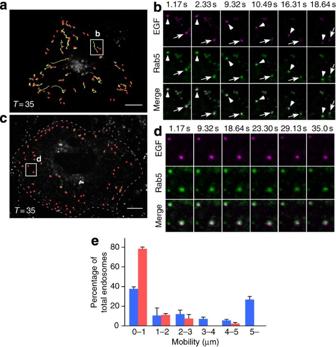Figure 4: Depletion of LRRK1 inhibits the motility of EGF-containing early endosomes. (a) Images representing GFP-Rab5-positive endosomes containing Alexa 647-EGF (red circles) and tracks (yellow). HeLa S3 cells treated with control siRNA were transfected with GFP-Rab5, pulse-labelled with Alexa 647-EGF. Movement of GFP-Rab5-positive endosomes containing Alexa 647-EGF was observed by time-lapse confocal fluorescence microscopy and analysed using the 'Manual Tracking' Image J plug-in. Imaging started at 15 min after the initial exposure to Alexa 647-EGF, with frames captured at 1.165 s intervals for 35 s. Scale bar, 10 μm. (b) Stills from control cells (the boxed region ina). Arrowheads and arrows indicate the movement of GFP-Rab5-positive endosome containing Alexa 647-EGF. (c) Images representing GFP-Rab5-positive endosomes containing Alexa 647-EGF (red circles) and tracks (yellow). HeLa S3 cells treated with LRRK1 siRNA (Stealth#1) were transfected with GFP-Rab5, pulse-labelled with Alexa 647-EGF. Movement of GFP-Rab5-positive endosomes containing Alexa 647-EGF was observed by time-lapse confocal fluorescence microscopy and analysed using the 'Manual Tracking' Image J plug-in. Imaging started at 15 min after the initial exposure to Alexa 647-EGF, with frames captured at 1.165 s intervals for 35 s. Scale bar, 10 μm. (d) Stills from LRRK1-depleted cells (the boxed region inc). (e) A mobility histogram of randomly selected Rab5- and EGF-double-positive endosomes from control (blue) or LRRK1-depleted cells (red). Mobility is defined as the distance of the trajectory of endosomes during the 35 s observation period, quantified using the 'Manual Tracking' Image J plug-in. Values reflect the mean s.d. of five independent experiments, with an average of 30 Rab5- and EGF-double-positive endosomes scored per experiment. Figure 4: Depletion of LRRK1 inhibits the motility of EGF-containing early endosomes. ( a ) Images representing GFP-Rab5-positive endosomes containing Alexa 647-EGF (red circles) and tracks (yellow). HeLa S3 cells treated with control siRNA were transfected with GFP-Rab5, pulse-labelled with Alexa 647-EGF. Movement of GFP-Rab5-positive endosomes containing Alexa 647-EGF was observed by time-lapse confocal fluorescence microscopy and analysed using the 'Manual Tracking' Image J plug-in. Imaging started at 15 min after the initial exposure to Alexa 647-EGF, with frames captured at 1.165 s intervals for 35 s. Scale bar, 10 μm. ( b ) Stills from control cells (the boxed region in a ). Arrowheads and arrows indicate the movement of GFP-Rab5-positive endosome containing Alexa 647-EGF. ( c ) Images representing GFP-Rab5-positive endosomes containing Alexa 647-EGF (red circles) and tracks (yellow). HeLa S3 cells treated with LRRK1 siRNA (Stealth#1) were transfected with GFP-Rab5, pulse-labelled with Alexa 647-EGF. Movement of GFP-Rab5-positive endosomes containing Alexa 647-EGF was observed by time-lapse confocal fluorescence microscopy and analysed using the 'Manual Tracking' Image J plug-in. Imaging started at 15 min after the initial exposure to Alexa 647-EGF, with frames captured at 1.165 s intervals for 35 s. Scale bar, 10 μm. ( d ) Stills from LRRK1-depleted cells (the boxed region in c ). ( e ) A mobility histogram of randomly selected Rab5- and EGF-double-positive endosomes from control (blue) or LRRK1-depleted cells (red). Mobility is defined as the distance of the trajectory of endosomes during the 35 s observation period, quantified using the 'Manual Tracking' Image J plug-in. Values reflect the mean s.d. of five independent experiments, with an average of 30 Rab5- and EGF-double-positive endosomes scored per experiment. Full size image The role of Roc and kinase domains in EGFR trafficking Ras proteins switch between an inactive GDP-bound state and an active GTP-bound state and only the latter interacts with its downstream effectors. Among the best characterized downstream effectors of Ras are the MAPKKKs [21] . Members of the ROCO protein family contain a Ras GTPase-like (Roc) domain and a MAPKKK domain ( Fig. 1b ). The Roc domain likely serves as a molecular switch, regulating kinase activity by cycling between GDP-bound and GTP-bound states [22] , [23] , [24] . To test whether the Roc domain of LRRK1 also regulates its kinase activity, we generated LRRK1(S625N) ( Fig. 1b ), in which Ser-625 in the Roc domain of LRRK1 has been mutated to Asn, on the basis of homology to Ras [25] . We confirmed that the LRRK1(S625N) form lost the ability to bind to GTP sepharose ( Supplementary Fig. S10a ) and was defective in kinase activity, similar to a kinase-inactive LRRK1(K1243M) ( Fig. 1b ; Supplementary Fig. S10b ). These results are consistent with a model wherein the Roc domain regulates the activity of the kinase domain. We next examined whether LRRK1(K1243M) or LRRK1(S625N) could rescue the defect in EGFR trafficking caused by LRRK1 knockdown. A large fraction of EGF dissociated from early endosomes 20 min after EGF-Rh stimulation in control siRNA-treated cells ( Supplementary Fig. S11a ), whereas the EGF remained localized in early endosomes in LRRK1 siRNA-treated cells ( Supplementary Fig. S11b ), as evidenced by their co-localization with EEA1. Expression of siRNA-resistant wild-type GFP-LRRK1 in LRRK1-depleted cells decreased co-localization of EGF with EEA1 and somewhat enhanced the transport of EGF towards the cell centre at 20 min after EGF-Rh stimulation ( Supplementary Fig. S11c ), suggesting that EGF was localized in late endosomes. When siRNA-resistant GFP-LRRK1(K1243M) or GFP-LRRK1(S625N) was reintroduced into LRRK1-depleted cells, most of the EGF remained co-localized with EEA1 even after a chase of 20 min ( Supplementary Fig. S11d,e ). Furthermore, we found that siRNA-resistant wild-type GFP-LRRK1, but not GFP-LRRK1(K1232M), was able to rescue the movement of EGF in LRRK1-depleted cells ( Supplementary Fig. S12 ). These results suggest that the kinase function of LRRK1 is required for the transport of EGF/EGFR from early to late endosomes. The relationship between LRRK1 and the ESCRT-0 complex Trafficking of EGF/EGFR in early endosomes is initiated by the interaction of ubiquitinated EGFR with components of the ESCRT-0 complex, STAM and Hrs [6] , [7] , [8] , [9] , [10] . To determine whether the effect of LRRK1 on EGFR trafficking involves these endosomal sorting components, we examined the interaction of LRRK1 with STAM and Hrs. COS7 cells were transfected with GFP-LRRK1 and stimulated with EGF. Coimmunoprecipitation experiments revealed that LRRK1 associated with endogenous STAM1 and that this interaction was increased by EGF stimulation ( Fig. 5a ). Furthermore, we found that endogenous LRRK1 was coimmunoprecipitated with endogenous Hrs in an EGF stimulation-dependent manner ( Fig. 5b ). These results demonstrate that LRRK1 interacts with the ESCRT-0 complex in response to EGF stimulation. 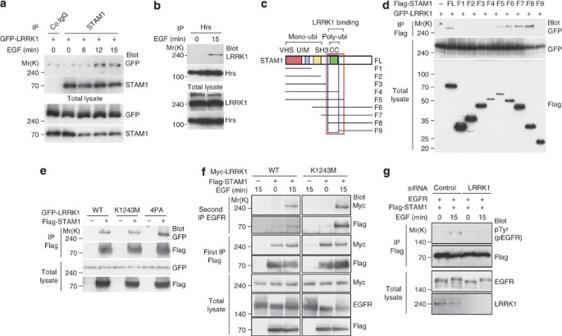Figure 5: LRRK1 interacts with the ESCRT-0 complex in response to EGF stimulation. (a) Association of LRRK1 with STAM1. COS7 cells were transfected with GFP-LRRK1, and stimulated with 100 ng per ml of EGF. Complex formation was detected by immunoprecipitation (IP) with anti-STAM1 antibodies, followed by immunoblotting (Blot) with anti-GFP antibodies. (b) Association of LRRK1 with Hrs. After 16 h of serum starvation, COS7 cells were stimulated with 100 ng per ml of EGF. Complex formation was detected by immunoprecipitation (IP) with anti-Hrs antibodies, followed by immunoblotting (Blot) with anti-LRRK1 antibodies. (c) Schematic diagram of STAM1 protein. Deletion constructs of STAM1 are shown below. (d) Interaction of STAM1 fragments with LRRK1. COS7 cells were co-transfected with Flag-STAM1 and GFP-LRRK1, as indicated. Complex formation was detected by immunoprecipitation (IP) with anti-Flag antibodies, followed by immunoblotting (Blot) with anti-GFP antibodies. (e) Interaction of STAM1 with LRRK1 variants. COS7 cells were co-transfected with GFP-LRRK1 (wild type, K1243M and 4PA mutants) and Flag-STAM1, as indicated. Complex formation was detected by immunoprecipitation (IP) with anti-Flag antibodies, followed by immunoblotting (Blot) with anti-GFP antibodies. (f) Both wild-type LRRK1 and LRRK1(K1243M) form a ternary complex with EGFR and STAM1 in response to EGF stimulation. COS7 cells were co-transfected with Myc-LRRK1 (wild type and the K1243 mutant) and Flag-STAM1, as indicated, stimulated with 100 ng per ml of EGF, and collected for the first immunoprecipitation (IP) with anti-Flag antibody-conjugated agarose. Thereafter, the immunocomplexes were eluted by 3xFlag peptide and subjected to the second immunoprecipitation (IP) with anti-EGFR antibodies, followed by immunoblotting (Blot) with anti-Myc and anti-Flag antibodies. (g) LRRK1 is required for the interaction between EGFR and STAM1. HeLa S3 cells treated with control or LRRK1 siRNA (Stealth#1) were co-transfected with EGFR and Flag-STAM1, and stimulated with 100 ng per ml of EGF. Complex formation was detected by immunoprecipitation (IP) with anti-Flag antibodies, followed by immunoblotting (Blot) with anti-phospho-tyrosine (pTyr) antibodies. Figure 5: LRRK1 interacts with the ESCRT-0 complex in response to EGF stimulation. ( a ) Association of LRRK1 with STAM1. COS7 cells were transfected with GFP-LRRK1, and stimulated with 100 ng per ml of EGF. Complex formation was detected by immunoprecipitation (IP) with anti-STAM1 antibodies, followed by immunoblotting (Blot) with anti-GFP antibodies. ( b ) Association of LRRK1 with Hrs. After 16 h of serum starvation, COS7 cells were stimulated with 100 ng per ml of EGF. Complex formation was detected by immunoprecipitation (IP) with anti-Hrs antibodies, followed by immunoblotting (Blot) with anti-LRRK1 antibodies. ( c ) Schematic diagram of STAM1 protein. Deletion constructs of STAM1 are shown below. ( d ) Interaction of STAM1 fragments with LRRK1. COS7 cells were co-transfected with Flag-STAM1 and GFP-LRRK1, as indicated. Complex formation was detected by immunoprecipitation (IP) with anti-Flag antibodies, followed by immunoblotting (Blot) with anti-GFP antibodies. ( e ) Interaction of STAM1 with LRRK1 variants. COS7 cells were co-transfected with GFP-LRRK1 (wild type, K1243M and 4PA mutants) and Flag-STAM1, as indicated. Complex formation was detected by immunoprecipitation (IP) with anti-Flag antibodies, followed by immunoblotting (Blot) with anti-GFP antibodies. ( f ) Both wild-type LRRK1 and LRRK1(K1243M) form a ternary complex with EGFR and STAM1 in response to EGF stimulation. COS7 cells were co-transfected with Myc-LRRK1 (wild type and the K1243 mutant) and Flag-STAM1, as indicated, stimulated with 100 ng per ml of EGF, and collected for the first immunoprecipitation (IP) with anti-Flag antibody-conjugated agarose. Thereafter, the immunocomplexes were eluted by 3xFlag peptide and subjected to the second immunoprecipitation (IP) with anti-EGFR antibodies, followed by immunoblotting (Blot) with anti-Myc and anti-Flag antibodies. ( g ) LRRK1 is required for the interaction between EGFR and STAM1. HeLa S3 cells treated with control or LRRK1 siRNA (Stealth#1) were co-transfected with EGFR and Flag-STAM1, and stimulated with 100 ng per ml of EGF. Complex formation was detected by immunoprecipitation (IP) with anti-Flag antibodies, followed by immunoblotting (Blot) with anti-phospho-tyrosine (pTyr) antibodies. Full size image To determine which regions are responsible for the LRRK1–STAM1 interaction, we constructed several deletion mutants of STAM1 ( Fig. 5c ). Coimmunoprecipitation assays showed that the coiled-coil domain of STAM1 was important for its interaction with LRRK1 ( Fig. 5d ). We next tested whether the kinase function of LRRK1 would affect its interaction with STAM1. We found that Flag-STAM1 coimmunoprecipitated with GFP-LRRK1(K1243M) ( Fig. 5e ), indicating that LRRK1 kinase activity is not required for its association with STAM1. In addition, the Grb2-binding-defective mutant GFP-LRRK1(4PA) was also able to associate with STAM1 ( Fig. 5e ), suggesting that different regions of LRRK1 interact with Grb2 and STAM1. We next examined whether LRRK1, EGFR and STAM1 exist in the same complex. Flag-STAM1 and Myc-LRRK1 or Myc-LRRK1(K1243M) were coexpressed in COS7 cells and ternary complex formation was investigated via two-step immunoprecipitation. Both Myc-LRRK1 and Myc-LRRK1(K1243M) were able to form a ternary complex with EGFR and STAM1 in response to EGF stimulation ( Fig. 5f ), indicating that LRRK1 kinase activity is not required for formation of this ternary complex. Given the results showing that LRRK1 interacts with EGFR and the ESCRT-0 complex, we reasoned that loss of LRRK1 should also result in decreased EGFR–ESCRT-0 complex formation. When cells were treated with LRRK1 siRNA, we observed a reduction in the EGF-dependent interaction of activated EGFR with Flag-STAM1 ( Fig. 5g ). Taken together, these results suggest that LRRK1, by interacting with both Grb2 and the Hrs–STAM1 complex simultaneously, functions as a scaffolding protein linking activated EGFR to the ESCRT-0 complex. To further evaluate the interaction between LRRK1 and STAM, we examined the potential co-localization of LRRK1 and STAM1 in early endosomes. Previous studies have revealed that Hrs accumulates in restricted microdomains on the endosome membrane, strongly co-localizing with clathrin [26] , [27] , [28] , [29] . By contrast, EEA1-containing regions of the endosome membrane are largely devoid of Hrs and clathrin. To study these endosomal microdomains, HeLa S3 cells were transfected with a constitutively active form of Rab5(Q79L), to increase the fusion rate of endosomes [30] . High Rab5 activity results in enlarged early endosomes on which microdomains can be easily distinguished by confocal immunofluorescence microscopy [26] , [27] , [29] , [31] . STAM1 co-localized strongly with clathrin on the enlarged endosomes ( Supplementary Fig. S13a ), whereas there was little co-localization of STAM1 and EEA1 ( Supplementary Fig. S13b ). These results suggest that STAM1 participates together with Hrs in the sorting of ubiquitinated cargo in clathrin-coated microdomains of early endosomes. GFP-LRRK1 was mainly distributed to the cytosol in the absence of EGF stimulation ( Fig. 6a ). However, LRRK1 localization was restricted to the enlarged endosomes of EGF-treated cells, and we could detect a certain degree of localization of GFP-LRRK1 to STAM1-positive microdomains ( Fig. 6b ). We also found that EGFR co-localized with STAM1 on Rab5(Q79L)-induced enlarged endosomes after EGF stimulation ( Fig. 6c ). To investigate whether LRRK1 is important for the recruitment of EGFR into STAM1-positive microdomains, we set out to study the relative localizations of EGFR and STAM1 in LRRK1-depleted cells. In such LRRK1-depleted cells, both EGFR and STAM1 could still be detected on endosomes. Interestingly, however, LRRK1-depleted endosomes appeared to show decreased co-localization of EGFR and STAM1 ( Fig. 6d ). Furthermore, this co-localization gradually increased at the later phase of EGF stimulation ( Fig. 6e ), indicating that LRRK1 depletion delays EGFR-STAM1 co-localization. We confirmed the effect of LRRK1 depletion on the co-localization of Alexa 647-EGF and STAM1 by three-dimensional reconstruction of confocal Z-stack images ( Supplementary Fig. S14 ). These results suggest that LRRK1 determines the efficiency of recruitment by serving as a scaffolding function on the endosomal membrane to restrict EGFR localization to STAM-positive microdomains. 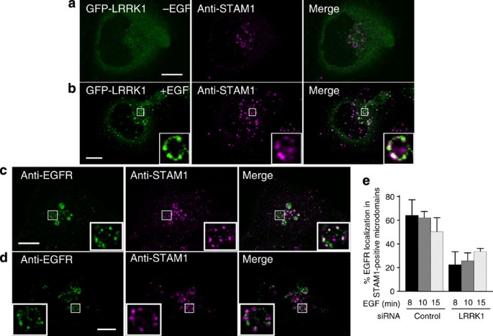Figure 6: Localization of LRRK1 and EGFR on STAM1-positive microdomains of early endosomes. (a,b) Localization of LRRK1 and STAM1 on enlarged endosomes. HeLa S3 cells were co-transfected with DsRed-Rab5(Q79L) and GFP-LRRK1, and stimulated without (a) or with (b) 100 ng per ml of EGF for 10 min. The cells were fixed and stained with anti-STAM1 antibodies and imaged by confocal microscopy. Experiments were conducted three times with similar results. Scale bar, 10 μm. (c,d) Effect of LRRK1 depletion on EGFR localization to STAM-positive microdomains of early endosomes. HeLa S3 cells treated with control (c) or LRRK1 siRNA (Stealth#1) (d) were transfected with GFP-Rab5(Q79L) and stimulated with 100 ng per ml of EGF for 10 min. The cells were fixed, stained with anti-EGFR and anti-STAM1 antibodies and imaged by confocal microscopy. The boxed regions indicate the Rab5(Q79L)-induced enlarged endosomes and are magnified in the inset. Scale bar, 10 μm. (e) Quantification of EGFR localization to STAM-positive microdomains of early endosomes. HeLa S3 cells treated with control or LRRK1 siRNA (Stealth#1) were transfected with GFP-Rab5(Q79L), and stimulated with 100 ng per ml of EGF for the indicated times. The cells were fixed, and stained with anti-EGFR and anti-STAM1 antibodies. Data show the percentage of STAM1-labelled EGFR-positive microdomains per endosomes. Values reflect the mean s.d. of three independent experiments, with an average of 15 cells (total 80 endosomes) scored per experiment. Figure 6: Localization of LRRK1 and EGFR on STAM1-positive microdomains of early endosomes. ( a , b ) Localization of LRRK1 and STAM1 on enlarged endosomes. HeLa S3 cells were co-transfected with DsRed-Rab5(Q79L) and GFP-LRRK1, and stimulated without ( a ) or with ( b ) 100 ng per ml of EGF for 10 min. The cells were fixed and stained with anti-STAM1 antibodies and imaged by confocal microscopy. Experiments were conducted three times with similar results. Scale bar, 10 μm. ( c , d ) Effect of LRRK1 depletion on EGFR localization to STAM-positive microdomains of early endosomes. HeLa S3 cells treated with control ( c ) or LRRK1 siRNA (Stealth#1) ( d ) were transfected with GFP-Rab5(Q79L) and stimulated with 100 ng per ml of EGF for 10 min. The cells were fixed, stained with anti-EGFR and anti-STAM1 antibodies and imaged by confocal microscopy. The boxed regions indicate the Rab5(Q79L)-induced enlarged endosomes and are magnified in the inset. Scale bar, 10 μm. ( e ) Quantification of EGFR localization to STAM-positive microdomains of early endosomes. HeLa S3 cells treated with control or LRRK1 siRNA (Stealth#1) were transfected with GFP-Rab5(Q79L), and stimulated with 100 ng per ml of EGF for the indicated times. The cells were fixed, and stained with anti-EGFR and anti-STAM1 antibodies. Data show the percentage of STAM1-labelled EGFR-positive microdomains per endosomes. Values reflect the mean s.d. of three independent experiments, with an average of 15 cells (total 80 endosomes) scored per experiment. Full size image LRRK1 modulates the ubiquitination status of STAM1 The sorting of ubiquitinated EGFR is initiated by the recognition of EGFR ubiquitin (Ub) moieties by the Ub-interacting motifs (UIMs) within Hrs and STAM [10] , [32] . Hrs and STAM themselves are also ubiquitinated [32] , [33] , and a recent study has suggested that intramolecular binding between UIMs and Ub prevents Hrs from binding in trans to ubiquitinated EGFR [32] . We therefore examined the effect of LRRK1 knockdown on the ubiquitination status of STAM1. We co-transfected HeLa S3 cells with Flag-STAM1 and HA-Ub. In control siRNA cells, we could detect weak ubiquitination of STAM1 and this ubiquitination was enhanced by EGF stimulation ( Fig. 7a ). Depletion of LRRK1 resulted in hyper-ubiquitination of STAM1 ( Fig. 7a ). Thus, depletion of LRRK1 results in the enhancement of Ub modification in STAM1. We then examined the effect of LRRK1 overexpression on the ubiquitination status of STAM1. We found that overexpression of LRRK1 inhibited ubiquitination of STAM1 ( Fig. 7b ). In addition, overexpression of kinase-negative LRRK1(K1243M) was able to inhibit STAM1 ubiquitination ( Fig. 7b ), suggesting that LRRK1 kinase activity is not necessary for this reaction. 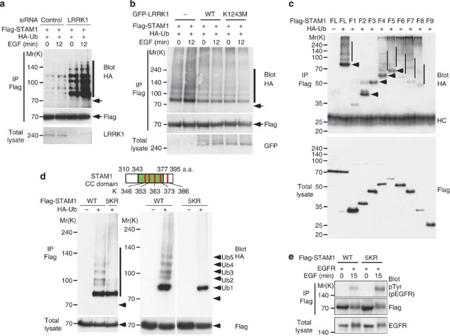Figure 7: LRRK1 modulates the ubiquitination status of STAM1. (a) Effect of LRRK1 depletion on the ubiquitination of STAM1. HeLa S3 cells treated with control or LRRK1 siRNA (Stealth#1) were co-transfected with Flag-STAM1 and HA-Ub, and stimulated with 100 ng per ml of EGF. Complexes immunoprecipitated (IP) with anti-Flag antibody were immunoblotted (Blot) with anti-HA antibodies. Arrows and line indicate the positions of the unmodified and ubiquitinated forms of Flag-STAM1, respectively. (b) Effect of LRRK1 overexpression on the ubiquitination of STAM1. COS7 cells were co-transfected with GFP-LRRK1 (wild type and the K1243 mutant), Flag-STAM1 and HA-Ub as indicated. Complexes immunoprecipitated (IP) with anti-Flag antibody were immunoblotted (Blot) with anti-HA antibodies. Arrows and line indicate the positions of the unmodified and ubiquitinated forms of Flag-STAM1, respectively. (c) Ubiquitination of STAM1. COS7 cells were co-transfected with Flag-STAM1 and HA-Ub as indicated. Complexes immunoprecipitated (IP) with anti-Flag antibodies were immunoblotted (Blot) with anti-HA antibodies. Arrowheads and lines indicate the positions of the monoubiquitinated and polyubiquitinated forms of Flag-STAM1, respectively. HC represents heavy chain. (d) Ubiquitination sites in STAM1. The lysine residues around the STAM1 coiled-coil domain (green) are shown. COS7 cells were co-transfected with Flag-STAM1 (wild type and the 5KR mutant) and HA-Ub as indicated. Complexes immunoprecipitated (IP) with anti-Flag antibodies were immunoblotted (Blot) with anti-HA antibodies. Arrows and line indicate the positions of the unmodified and ubiquitinated forms of Flag-STAM1, respectively. (e) Interaction between EGFR and STAM1(5KR). COS7 cells were co-transfected with Flag-STAM1 (wild type and the 5KR mutant) and EGFR as indicated, and stimulated with 100 ng per ml of EGF. Complex formation was detected by immunoprecipitation (IP) with anti-Flag antibodies, followed by immunoblotting (Blot) with anti-phospho-tyrosine (pTyr) antibodies. Figure 7: LRRK1 modulates the ubiquitination status of STAM1. ( a ) Effect of LRRK1 depletion on the ubiquitination of STAM1. HeLa S3 cells treated with control or LRRK1 siRNA (Stealth#1) were co-transfected with Flag-STAM1 and HA-Ub, and stimulated with 100 ng per ml of EGF. Complexes immunoprecipitated (IP) with anti-Flag antibody were immunoblotted (Blot) with anti-HA antibodies. Arrows and line indicate the positions of the unmodified and ubiquitinated forms of Flag-STAM1, respectively. ( b ) Effect of LRRK1 overexpression on the ubiquitination of STAM1. COS7 cells were co-transfected with GFP-LRRK1 (wild type and the K1243 mutant), Flag-STAM1 and HA-Ub as indicated. Complexes immunoprecipitated (IP) with anti-Flag antibody were immunoblotted (Blot) with anti-HA antibodies. Arrows and line indicate the positions of the unmodified and ubiquitinated forms of Flag-STAM1, respectively. ( c ) Ubiquitination of STAM1. COS7 cells were co-transfected with Flag-STAM1 and HA-Ub as indicated. Complexes immunoprecipitated (IP) with anti-Flag antibodies were immunoblotted (Blot) with anti-HA antibodies. Arrowheads and lines indicate the positions of the monoubiquitinated and polyubiquitinated forms of Flag-STAM1, respectively. HC represents heavy chain. ( d ) Ubiquitination sites in STAM1. The lysine residues around the STAM1 coiled-coil domain (green) are shown. COS7 cells were co-transfected with Flag-STAM1 (wild type and the 5KR mutant) and HA-Ub as indicated. Complexes immunoprecipitated (IP) with anti-Flag antibodies were immunoblotted (Blot) with anti-HA antibodies. Arrows and line indicate the positions of the unmodified and ubiquitinated forms of Flag-STAM1, respectively. ( e ) Interaction between EGFR and STAM1(5KR). COS7 cells were co-transfected with Flag-STAM1 (wild type and the 5KR mutant) and EGFR as indicated, and stimulated with 100 ng per ml of EGF. Complex formation was detected by immunoprecipitation (IP) with anti-Flag antibodies, followed by immunoblotting (Blot) with anti-phospho-tyrosine (pTyr) antibodies. Full size image We next attempted to narrow down the region(s) where STAM1 is ubiquitinated, using various deletion mutants of STAM1 ( Fig. 5c ). Ubiquitination assays revealed that the N-terminal Ub-binding domains (VHS and UIM) and the SH3 domain of STAM1 are important for monoubiquitination, and that the coiled-coil domain contains the majority of polyubiquitination sites in STAM1 ( Fig. 7c ). Thus, the coiled-coil domain of STAM1 is involved in both its interaction with LRRK1 and its ubiquitination, raising the possibility that LRRK1 inhibits STAM1 ubiquitination by associating with its coiled-coil domain. The coiled-coil domain in STAM1 has five lysine residues ( Fig. 7d ). To confirm the importance of the coiled-coil domain for STAM1 ubiquitination, we generated STAM1(5KR), in which all these five lysines have been mutated to arginines. STAM1(5KR) was impaired in polyubiquitination but not in monoubiquitination ( Fig. 7d ). These results suggest that the lysine residues in the coiled-coil domain of STAM1 are polyubiquitinated. The above results suggested that LRRK1 affects the interaction between EGFR and STAM1 by modulating the ubiquitination status of STAM1. Consistent with this, STAM1(5KR) showed an increase in its interaction with activated EGFR compared with wild-type STAM1 ( Fig. 7e ). Taken together, these results suggest that LRRK1 functions as a scaffolding protein linking activated EGFR to the ESCRT-0 complex by suppressing the polyubiquitination of STAM1. LRRK1 regulates sorting of EGF/EGFR into intraluminal vesicles of MVBs EGFR localized in clathrin-coated microdomains on endosomes is sorted into intraluminal vesicles (ILVs) within MVBs and delivered to lysosomes for degradation. We therefore examined whether LRRK1 knockdown affects the sorting of EGFR into ILVs of enlarged endosomes using three-dimensional reconstructions. In control siRNA-transfected cells, Alexa 647-EGF was translocated from the limiting membrane to ILVs of Rab5(Q79L)-induced enlarged endosomes at 30 min after EGF stimulation ( Fig. 8a ). In contrast, depletion of LRRK1 reduced the intraluminal transport of Alexa 647-EGF into enlarged endosomes ( Fig. 8b ). Line intensity profiles of individual endosomes clearly showed that most of the EGF was localized within the inner membranes in control cells ( Fig. 8c ), but were retained in the limiting membrane in LRRK1-depleted cells ( Fig. 8d ). Quantification of EGF labelling showed that about 66.2% of the labelling was localized to the inner membranes in cells treated with control siRNA, whereas only 16.7% showed this localization in cells treated with LRRK1 siRNA ( Fig. 8e ). These results demonstrate that LRRK1 is needed for sorting of EGF/EGFR into ILVs of MVBs. When siRNA-resistant, wild-type GFP-LRRK1 was expressed in LRRK1-depleted cells, the defect in the intraluminal transport of Alexa 647-EGF was partially rescued ( Fig. 8e ). However, expression of the siRNA-resistant, kinase-negative GFP-LRRK1(K1243M) was able to rescue the defect in EGF sorting in LRRK1-depleted cells ( Fig. 8e ), suggesting that LRRK1 kinase activity is not essential for this step. Thus, LRRK1 functions as a scaffold in this process, independent of its kinase activity. 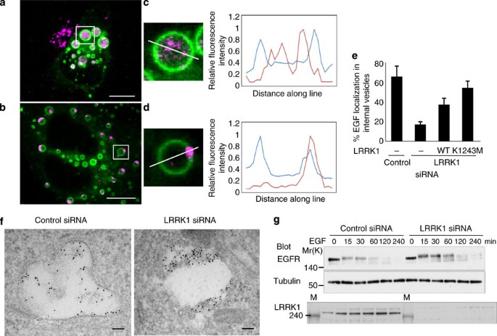Figure 8: Effects of LRRK1 depletion on localization of EGFR in MVBs and EGFR degradation. (a,b) Effect of LRRK1 depletion on EGFR sorting into the lumen of Rab5(Q79L)-induced enlarged endosomes. HeLa S3 cells treated with control (a) or LRRK1 siRNA (Stealth#1) (b) were transfected with DsRed-Rab5(Q79L) and stimulated with 100 ng per ml of Alexa 647-EGF for 30 min. The cells were fixed and imaged by confocal microscopy. Images are three-dimensional reconstructions from a series of confocal Z-stack images (0.3 μm-thick sections). Scale bar, 10 μm. (c,d) Confocal images from control (c; the boxed region ina) or LRRK1-depleted cells (d; the boxed region inb) show individual enlarged endosomes. Areas of co-localization are shown by line intensity profiles. (e) Quantification of Alexa 647-EGF localization into the lumen of Rab5(Q79L)-induced enlarged endosomes. Cells treated with control or LRRK1 siRNA (Stealth#1) were co-transfected with DsRed-Rab5(Q79L) and siRNA-resistant GFP-LRRK1 (wild type and the K1243 M mutant), as indicated. Cells were stimulated with 100 ng per ml of Alexa 647-EGF for 30 min and then fixed. Data are presented as percentages of Alexa 647-EGF localization into the lumen of enlarged endosomes out of the total number of Rab5(Q79L)-induced enlarged endosomes (diameter; >1 μm). Values reflect the mean s.d. of three independent experiments, with an average of 15 cells (total 100 endosomes) scored per experiment. (f) HeLa S3 cells were treated with control or LRRK1 siRNA (Stealth#1). After 16 h of serum starvation, cells were incubated with anti-EGFR antibodies (LA-22) for 2 h at 37°C, followed by goat anti-mouse IgM antibodies conjugated to 10 nm gold for 1 h at 37°C. After washing to remove antibodies from the medium, the cells were stimulated with EGF for 10 min and then fixed. The localization of EGFR was examined by silver-enhanced immunogold electron microscopy. Scale bar, 100 nm. (g) HeLa S3 cells treated with control or LRRK1 siRNA (Stealth#1) were transfected with EGFR. After 16 h of serum starvation, cells were stimulated with 100 ng per ml of EGF. Cell lysates were immunoblotted with indicated antibodies. Tubulin serves as a loading control. Figure 8: Effects of LRRK1 depletion on localization of EGFR in MVBs and EGFR degradation. ( a , b ) Effect of LRRK1 depletion on EGFR sorting into the lumen of Rab5(Q79L)-induced enlarged endosomes. HeLa S3 cells treated with control ( a ) or LRRK1 siRNA (Stealth#1) ( b ) were transfected with DsRed-Rab5(Q79L) and stimulated with 100 ng per ml of Alexa 647-EGF for 30 min. The cells were fixed and imaged by confocal microscopy. Images are three-dimensional reconstructions from a series of confocal Z-stack images (0.3 μm-thick sections). Scale bar, 10 μm. ( c , d ) Confocal images from control ( c ; the boxed region in a ) or LRRK1-depleted cells ( d ; the boxed region in b ) show individual enlarged endosomes. Areas of co-localization are shown by line intensity profiles. ( e ) Quantification of Alexa 647-EGF localization into the lumen of Rab5(Q79L)-induced enlarged endosomes. Cells treated with control or LRRK1 siRNA (Stealth#1) were co-transfected with DsRed-Rab5(Q79L) and siRNA-resistant GFP-LRRK1 (wild type and the K1243 M mutant), as indicated. Cells were stimulated with 100 ng per ml of Alexa 647-EGF for 30 min and then fixed. Data are presented as percentages of Alexa 647-EGF localization into the lumen of enlarged endosomes out of the total number of Rab5(Q79L)-induced enlarged endosomes (diameter; >1 μm). Values reflect the mean s.d. of three independent experiments, with an average of 15 cells (total 100 endosomes) scored per experiment. ( f ) HeLa S3 cells were treated with control or LRRK1 siRNA (Stealth#1). After 16 h of serum starvation, cells were incubated with anti-EGFR antibodies (LA-22) for 2 h at 37°C, followed by goat anti-mouse IgM antibodies conjugated to 10 nm gold for 1 h at 37°C. After washing to remove antibodies from the medium, the cells were stimulated with EGF for 10 min and then fixed. The localization of EGFR was examined by silver-enhanced immunogold electron microscopy. Scale bar, 100 nm. ( g ) HeLa S3 cells treated with control or LRRK1 siRNA (Stealth#1) were transfected with EGFR. After 16 h of serum starvation, cells were stimulated with 100 ng per ml of EGF. Cell lysates were immunoblotted with indicated antibodies. Tubulin serves as a loading control. Full size image We confirmed the above immunofluorescence data by electron microscopy. Silver-enhanced gold particles revealed the presence of endogenous EGFR associated with both the limiting membrane and ILVs of MVBs in control cells, whereas most of the EGFR was still located on the limiting membrane of MVBs in LRRK1-depleted cells ( Fig. 8f ). We next asked whether LRRK1 could also affect EGFR degradation. Although EGF stimulation normally causes the degradation of EGFR, we observed stabilization of activated EGFR in cells treated with LRRK1 siRNA ( Fig. 8g ). These results suggest that LRRK1 is required for EGFR sorting into the degradative pathway. EGFR targeted for lysosomal degradation is delivered to MVBs by a highly specialized process that begins with receptor ubiquitination and sequestration by elements of the ESCRT complex on the surface of early endosomes [6] , [7] , [8] , [9] , [10] . Endosomal sorting of ubiquitinated EGFR is initiated by ESCRT-0, which is composed of Hrs and STAM [6] , [7] , [8] , [9] , [10] . It has been proposed that Hrs and STAM can concentrate ubiquitinated cargo on clathrin-coated microdomains of early endosomes and link the cargo with the subsequent ESCRT machinery that is required for proper sorting [27] , [29] , [31] . In this study, we show that LRRK1 is required for EGFR transport from early to late endosomes. Our results demonstrate that LRRK1 forms a complex with EGFR via Grb2 and associates with STAM and Hrs in response to ligand stimulation. Furthermore, we find that knockdown of LRRK1 disrupts the recruitment of EGFR to STAM1-positive microdomains of early endosomes, leading to the inhibition of EGFR sorting to the inner vesicles of MVBs. LRRK1 may function as a scaffolding protein between ubiquitinated EGFR and the Hrs–STAM1 complex. Consistent with this possibility, EGFR, LRRK1 and STAM1 can form a ternary complex in response to EGF stimulation, and knockdown of LRRK1 disrupts the interaction of EGFR with STAM1. In addition, our data suggest a mechanism whereby LRRK1 modulates the ubiquitination status of STAM1 by direct interaction. It is likely that ubiquitination of STAM1, which leads to intramolecular binding within STAM1, inhibits its ability to interact with ubiquitinated EGFR. Therefore, LRRK1 promotes complex formation between activated EGFR and STAM1 by decreasing the ubiquitination of STAM1. Our findings suggest that LRRK1 might function as a cargo-specific factor that efficiently links the activated EGFR to the ESCRT machinery. Remarkably, we find that the motility of EGF-containing early endosomes is diminished dramatically by LRRK1 knockdown. We demonstrate that LRRK1 kinase activity is required for the transport of EGFR-containing early endosomes from the periphery to the centre. Recent studies have shown that early endosomes move towards the cell centre as they mature [18] , [20] . The movement of early endosomes is mediated by cytoplasmic dynein, a minus end-directed microtubule motor [19] , [34] . LRRK1 might thus be involved in the regulation of dynein-dependent transport of EGF-containing early endosomes. Interestingly, in a screen for LRRK1-binding proteins, we have identified NudC and CLIP-170, which are involved in dynein-mediated processes [35] , [36] . Thus, LRRK1 might regulate the motility of EGF-containing early endosomes by phosphorylating these candidates. Because excessive or inappropriate signalling by activated EGFR is associated with the development of a broad range of human cancers, the spatiotemporal regulation of EGFR trafficking by LRRK1 is likely to be important for the maintenance of cellular homoeostasis. Identification of specific LRRK1 targets involved in the regulation of EGFR trafficking in early endosomes will be necessary. Further analysis of LRRK1 function may shed new light on the molecular mechanisms regulating the intracellular trafficking of EGFR, and thus the spatiotemporal control of EGFR signalling. Plasmids and mutations Human LRRK1 cDNA was subcloned into vector pGFP-C1 (Clontech), pCMV or pCS2. LRRK1(4PA), LRRK1(K1243M) and LRRK1(S625N) were generated using the QuickChange Site-Directed Mutagenesis Kit according to the manufacturer's protocol (Stratagene). siRNA-resistant LRRK1 was generated by mutating the target sequence of the LRRK1 siRNA (5′-GCAGGAACAGGAAAGTCACCATTTA-3′) into 5′-GTCGAAATCGAAAAGTCACCATTTA-3′. Human LRRK2 (Park8) cDNA was subcloned into vector pCMV. HA-Grb2(P49L), HA-Grb2(S90N), HA-Grb2(G203R) and HA-Grb2(P49L/G203R) were generated using the mutagenesis kit described above and subcloned into vector pSRα [37] . Human Rab5 and Rab7 were subcloned into vector pGFP-C1 or pDsRed-C1 (Clontech; catalogue number 632466), and Rab5(Q79L) was generated using the mutagenesis kit described above. pDsRed-C1 produces the monomer form of DsRed. Deletion constructs of STAM1 were generated by PCR-based mutagenesis and subcloned into pCMV-Flag. Antibodies and reagents Rabbit antibodies against LRRK1 were produced by MBL (Medical and Biological Laboratories) by injecting rabbits with synthetic peptides corresponding to residues 1767–1783 and 1848–1865 of LRRK1 coupled to keyhole limpet haemocyanin. Antibodies and their suppliers were as follows: anti-HA (16B12, Babco); anti-Flag (M2, Sigma); anti-Myc (9E10, Santa Cruz Biotechnology); anti-GFP (JL-8 or Full-length polyclonal antibody, Clontech); anti-phospho-Tyr (4G10, Upstate Biotechnology); anti-EGFR (SC-03, Santa Cruz Biotechnology, LA22, Upstate Biotechnology or 6F1, MBL); anti-Grb2 (SC-23, Santa Cruz Biotechnology); anti-EEA1 (Clone 14, BD Transduction Laboratories); anti-STAM1 (H-175, Santa Cruz Biotechnology); anti-Hrs (A-5, Alexis Biochemicals); anti-clathrin (clone 23, BD Transduction Laboratories); anti-Tubulin (B-5-1-2, Sigma); Goat anti-mouse IgM conjugated to 10 nm gold (BBinternational). EGF-Rh and Alexa647-EGF were purchased from Molecular Probes and human recombinant EGF from TOYOBO. Cell cultures and transfections HeLa, HeLa S3, HEK293 and COS7 cells were cultured in Dulbecco's modified Eagle's medium containing 10% fetal bovine serum. These cells were split on 35-mm, 60-mm or 100-mm dishes at 2×10 5 , 5×10 5 or 2×10 6 cells per dish, respectively. After 19 h, cells were transfected using RNAi MAX (Invitrogen) or FuGENE 6 reagent (Roche Applied Science) according to the manufacturer's protocol. Immunoprecipitation For immunoprecipitation, cells were lysed in RIPA buffer containing 50 mM Tris-HCl (pH 7.4), 150 mM NaCl, 0.25% deoxycholic acid, 1% NP-40, 1 mM EDTA, 2 mM dithiothreitol, 1 mM phenylmethylsulphonyl fluoride, phosphatase inhibitor cocktail 2 (Sigma) and protease inhibitor cocktail (Sigma), followed by centrifugation at 15,000 g for 15 min. The supernatant was added to 10 μl (bed volume) of protein G sepharose beads (GE Healthcare) or Dynabeads protein G (Invitrogen) with the indicated antibodies and rotated for 2 h at 4°C or for 10 min at room temperature. The beads were washed three times with ice-cold phosphate-buffered saline and subjected to immunoblotting or kinase assays. Immunoblotting After the extracts were subjected to SDS–polyacrylamide gel electrophoresis (SDS–PAGE), proteins were transferred to polyvinylidene difluoride membrane (Hybond-P, GE Healthcare). Membranes were incubated with indicated antibodies using the SNAP i.d. system (Millipore). Immunoreactive bands were detected by an HRP chemiluminescent substrate reagent kit (Novex ECL, Invitrogen). In vitro autophosphorylation assay Immunocomplex kinase reactions of GFP-LRRK1, GFP-LRRK1(K1243M) or GFP-LRRK1(S625N) were performed in a final volume of 20 μl containing 20 mM Tris-HCl (pH7.4), 5 mM EGTA, 15 mM MgCl2, 5 μCi of [γ- 32 P]ATP. Samples were incubated for 20 min at 30°C. Reactions were terminated by the addition of Laemmli sample buffer and boiling. GFP-LRRK1, GFP-LRRK1(K1243M) or GFP-LRRK1(S625N) was resolved by SDS–PAGE. Autophosphorylation of LRRK1 was detected by autoradiography. RNA interference siRNA targeted against human LRRK1, human Grb2 and negative control siRNAs were purchased from Invitrogen and Ambion. Stealth siRNA (Stealth#1) for human LRRK1 (target sequence: 3165gcaggaacaggaaagtcaccattta TT), Silencer Validated siRNA (Ambion#1) for human LRRK1 (target sequence: 5493ggaatcactcactgactac TT) and Custom siRNA for human Grb2 (target sequence: 607catgtttccccgcaattat TT) [15] were used. Annealed siRNAs were transfected using RNAiMAX (Invitrogen). The transfected cells were analysed 72 h after transfection. For immunofluorescence experiments, cells were transfected with control siRNA, Grb2 siRNA or LRRK1 siRNA using RNAiMAX, incubated overnight and then transfected with GFP-LRRK1, GFP-Rab5, DsRed-Rab7, GFP-Rab5(Q79L) or DsRed-Rab5(Q79L) in the indicated combinations, using FuGENE 6 reagent (Roche Applied Science). GTP-binding studies Cells were lysed at 48 h post transfection in lysis buffer G (100 mM Tris-HCl pH 7.5, 50 mM KCl, 1 mM EDTA, 0.1 mM dithiothreitol, 5 mM MgCl2, 1% Triton X-100) containing phosphatase inhibitor cocktail and protease inhibitor cocktail (Sigma) for 10 min on ice, and lysates were clarified by centrifugation at 15,000 g for 10 min at 4°C. Supernatants were incubated with 20 μl of GTP-sepharose bead suspension (Sigma) by rotating at 4°C for 2 h and then sequentially pelleted and washed three times with 1 ml PBS. For guanine nucleotide competition experiments, GTP (Sigma) was added to a final concentration of 2 mM, and incubation was continued for a further 60 min at 4°C followed by washing. Precipitated proteins were resolved by SDS–PAGE and immunoblotted with anti-GFP antibodies. Fluorescence microscopy For immunofluorescence microscopy, cells grown on coverslips were treated, as indicated, and then fixed in 4% paraformaldehyde, permeabilized in 0.5% Triton X-100 and incubated with primary and secondary antibodies. Primary antibodies were anti-EEA1 at 1:100, anti-EGFR at 1:100, anti-STAM1 at 1:250 and anti-clathrin at 1:100. Secondary antibodies were Alexa-Fluor 647 goat anti-mouse IgG, Alexa-Fluor 555 goat anti-mouse IgG and Alexa-Fluor 488 goat anti-mouse IgG (Molecular Probes). Confocal microscopy was performed using an Olympus FV1000 microscope. For live-cell fluorescence microscopy, cells were grown in 35-mm plastic-bottomed dishes. Time-lapse images were obtained with a laser scanning confocal microscope (FV1000; Olympus). Tracking of GFP-Rab5- and A647-EGF-positive endosomes was conducted using the 'Manual Tracking' Image J plug-in (National Institutes of Health). Conventional electron microscopy Conventional electron microscopy was performed as described previously [38] . In brief, cells were fixed in 2.5% glutaraldehyde in 0.1 M sodium phosphate buffer at pH 7.4 for 20 min. The specimens were postfixed in buffer containing 1% OsO 4 , dehydrated in a series of graded ethanol solutions and embedded in epoxy resin. Ultrathin sections were collected and stained with uranylacetate and lead citrate and observed under an H7600 transmission electron microscope (Hitachi). How to cite this article: Hanafusa, H. et al . Leucine-rich repeat kinase LRRK1 regulates endosomal trafficking of the EGF receptor. Nat. Commun. 2:158 doi: 10.1038/ncomms1161 (2011).